LGALS3BP regulates centriole biogenesis and centrosome hypertrophy in cancer cells Centrosome morphology and number are frequently deregulated in cancer cells. Here, to identify factors that are functionally relevant for centrosome abnormalities in cancer cells, we established a protein-interaction network around 23 centrosomal and cell-cycle regulatory proteins, selecting the interacting proteins that are deregulated in cancer for further studies. One of these components, LGALS3BP, is a centriole- and basal body-associated protein with a dual role, triggering centrosome hypertrophy when overexpressed and causing accumulation of centriolar substructures when downregulated. The cancer cell line SK-BR-3 that overexpresses LGALS3BP exhibits hypertrophic centrosomes, whereas in seminoma tissues with low expression of LGALS3BP, supernumerary centriole-like structures are present. Centrosome hypertrophy is reversed by depleting LGALS3BP in cells endogenously overexpressing this protein, supporting a direct role in centrosome aberration. We propose that LGALS3BP suppresses assembly of centriolar substructures, and when depleted, causes accumulation of centriolar complexes comprising CPAP, acetylated tubulin and centrin. The centrosome in animal cells consists of at least 300 different proteins that were identified via biochemical, bioinformatic, genetic, functional and localization studies [1] , [2] . The main structural feature of the centrosome is the centriole pair surrounded by pericentriolar material (PCM). Scaffold proteins [3] , [4] have been proposed to serve as a binding matrix for the microtubule nucleation complex, the γ-tubulin ring complex that comprises at least nine different proteins [5] . The central component of this complex is the evolutionarily highly conserved γ-tubulin (TUBG1) [6] that forms together with TUBGCP2 and TUBGCP3 the γ-tubulin small complex (γ-TuSC) [7] . γ-TuSC is critical for microtubule nucleation, spindle organization and centrosome integrity [8] . Several comprehensive approaches have identified new centrosomal components and their function: genome-wide RNA interference (RNAi) screening combined with automated microscopy [9] , [10] , [11] , proteomics of the human interphase centrosome [12] , the Drosophila mitotic centrosome [13] , the basal body in Chlamydomonas [14] and bioinformatics studies [15] . Highly conserved proteins that have a role in ciliopathies and in molecular pathways of centrosome and centriole assembly have been defined through these and follow-up approaches [16] , [17] . Centrosome function, replication, segregation and structure maintenance depends on regulatory proteins of cell cycle and other cellular signalling pathways [18] , [19] , [20] , [21] . In cancer cells, centrosome morphology and number are frequently dysregulated [22] , [23] . The origin of most of these aberrations on a molecular level is unclear as mutations in centrosomal genes are rare [24] , [25] . However, there is a correlation between centrosome defects and dysregulation of cell-cycle regulatory kinases, inactivation of tumour suppressors and activated oncogenes [26] , [27] , [28] . Alternatively, these abnormalities could also be the result of overexpression of centrosomal proteins, cytokinesis failure, centrosome overduplication or cell fusion [25] . Here we established a protein–protein interaction network of some of the major centrosomal proteins to identify potential functional dependencies relating to centrosome abnormalities detected in cancer cells. Tandem affinity purification mass spectrometry (TAP-MS) identified three major hubs in the centrosome interaction network with at least 10 different interaction partners for TUBG1, TUBGCP3 and CEP250. We functionally characterized in human somatic proliferating cells, cancer cell models and patient tissues an interaction partner of TUBGCP3—the centriole-associated protein LGALS3BP—that we found to have a role for centriole biogenesis and cause PCM hypertrophy when dysregulated in cancer cells. Although higher levels of LGALS3BP expression lead to the dispersion of PCM, depletion results in the generation of multiple centriolar structures. The PCM hypertrophy- and accumulation of centriolar structure-phenotypes correlate directly with centrosome morphology aberrations in cancer cells and patient tissues with deregulated levels of LGALS3BP. Indeed, knockdown of LGALS3BP in the cancer cell line SK-BR-3 that exhibits hypertrophic centrosomes and has highly elevated levels of this protein recovers a more normal centrosome phenotype, thus suggesting a causal link between LGALS3BP dysregulation and the centrosome abnormalities demonstrated by high-grade cancer cells. An interaction network identifies new centrosomal components Our study aimed at identifying biochemical and functional protein networks within the centrosome and links between the centrosome and regulatory or signalling proteins relating to structural and functional centrosome aberrations in cancer. For this purpose, we expressed 23 centrosomal and cell-cycle regulatory proteins as bait proteins in human embryonic kidney cells (HEK293) for TAP-MS. The identified 2,703 (1,814 unique, 1,560 without auto-interactions and contaminations) protein interactions were integrated into a large protein–protein interaction network ( Supplementary Data 1 ) and a focused protein–protein interaction network among centrosomal proteins ( Fig. 1a ). The multiplicity of interactions with γ-TuSC components ( Supplementary Data 1 ) suggests that a series of proteins has a function that is closely related to γ-TuSC, possibly modulating its function or interactions with other centrosomal components. 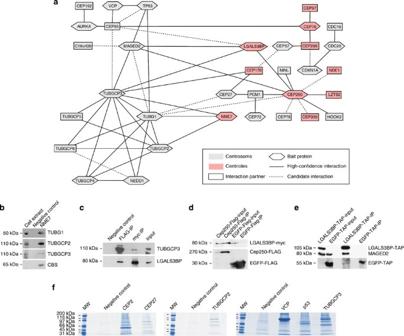Figure 1: A centrosomal protein-interaction network identifies new centrosomal proteins. (a) Protein–protein interaction subnetwork derived from the complete TAP interaction network (Supplementary Data 1) that displays known, newly identified or newly localized centrosome proteins (LGALS3BP and MAGED2). Interactions are represented as edges between bait proteins and their interaction partners. The bait proteins are displayed as hexagons, centrosomal proteins are coloured in grey and centriolar proteins in red. High-confidence interactions (Mascot score of the prey protein >50, at least two identified peptides) are shown with solid lines, and candidate interactions (Mascot score >24) are shown with dotted lines. (b,c) The protein–protein interactions of the main targets were validated by either reverse TAP (b) or co-immunoprecipitation (c). (b) The interactions of NME7 with TUBG1, TUBGCP2 and TUBGCP3 were confirmed by reverse TAP. The bait protein NME7 is identified through its TAP-tag moiety calmodulin-binding site (CBS). The cell extract was used as a positive western blotting control for the identification of the three NME7-interacting proteins. (c) The interaction between LGALS3BP and TUBGCP3 was confirmed by co-immunoprecipitation after co-expression of FLAG-TUBGCP3 and Myc-LGALS3BP in HEK293 cells. (d) The interactions between Myc-tagged LGALS3BP and a Flag-tagged CEP250 fragment co-expressed in HEK293 cells were confirmed by Flag-immunoprecipitation. Flag-tagged EGFP co-expressed with Myc-tagged LGALS3BP were used as negative control of the Flag-IP. (e) Endogenous MAGED2 interacts with TAP-tagged LGALS3BP. TAP-tagged EGFP was used as a negative control in the TAP experiments. (f) Examples of Coomassie stained 1-cm long SDS–PAGE gels of TAP eluates of centrosome-related bait proteins. The samples show the complexity of centrosomal protein-interacting proteins subjected to MS identification, in comparison with control samples (mock purification). Figure 1: A centrosomal protein-interaction network identifies new centrosomal proteins. ( a ) Protein–protein interaction subnetwork derived from the complete TAP interaction network ( Supplementary Data 1 ) that displays known, newly identified or newly localized centrosome proteins (LGALS3BP and MAGED2). Interactions are represented as edges between bait proteins and their interaction partners. The bait proteins are displayed as hexagons, centrosomal proteins are coloured in grey and centriolar proteins in red. High-confidence interactions (Mascot score of the prey protein >50, at least two identified peptides) are shown with solid lines, and candidate interactions (Mascot score >24) are shown with dotted lines. ( b , c ) The protein–protein interactions of the main targets were validated by either reverse TAP ( b ) or co-immunoprecipitation ( c ). ( b ) The interactions of NME7 with TUBG1, TUBGCP2 and TUBGCP3 were confirmed by reverse TAP. The bait protein NME7 is identified through its TAP-tag moiety calmodulin-binding site (CBS). The cell extract was used as a positive western blotting control for the identification of the three NME7-interacting proteins. ( c ) The interaction between LGALS3BP and TUBGCP3 was confirmed by co-immunoprecipitation after co-expression of FLAG-TUBGCP3 and Myc-LGALS3BP in HEK293 cells. ( d ) The interactions between Myc-tagged LGALS3BP and a Flag-tagged CEP250 fragment co-expressed in HEK293 cells were confirmed by Flag-immunoprecipitation. Flag-tagged EGFP co-expressed with Myc-tagged LGALS3BP were used as negative control of the Flag-IP. ( e ) Endogenous MAGED2 interacts with TAP-tagged LGALS3BP. TAP-tagged EGFP was used as a negative control in the TAP experiments. ( f ) Examples of Coomassie stained 1-cm long SDS–PAGE gels of TAP eluates of centrosome-related bait proteins. The samples show the complexity of centrosomal protein-interacting proteins subjected to MS identification, in comparison with control samples (mock purification). Full size image The validity of our results was confirmed by the identification of known interaction partners ( Supplementary Data 1 ), by conducting reverse TAP of the TUBG1, TUBGCP2 and TUBGCP3 interaction partner NME7 ( Fig. 1b ), through bidirectional co-immunoprecipitation of LGALS3BP and TUBGCP3 ( Fig. 1c ) and confirmation of the interactions of TAP-tagged LGALS3BP with endogenous MAGED2 and a Flag-tagged CEP250 expression construct with Myc-tagged LGALS3BP ( Fig. 1d ). The complexity of samples and enrichment is documented in the Coomassie gel analysis of the TAP samples before MS analysis ( Fig. 1f ). Furthermore, we added five different confidence scores to the list of interactions enabling a better assessment of the interaction’s significance: the first score indicates if the interaction was reciprocal, that is, if it was found in both directions within the TAP experiments. The next four scores were obtained by the IntScore web tool [29] : semantic similarity (a value between 0 and 1) regarding the gene ontology categories ‘biological process’ and ‘cellular compartment’; next, if the interaction partners are part of the same pathway; and finally, if the interaction was already described in the literature before. The latter two scores are calculated on the basis of ConsensusPathDB [30] , a database that integrates 31 different public pathway databases. In summary, a large fraction of the network (1,210 of 1,565 interactions=77.3%) was confirmed by at least one of these five scores. 189 interactions (12.1%) were confirmed by three or more scores. To define a protein–protein interaction network among centrosomal proteins ( Fig. 1a ), we selected from the large cohort of TAP interactions only known centrosomal proteins plus newly identified MAGED2 and LGALS3BP. Major hubs of this network are TUBG1 (10 interactions), TUBGCP3 (11 interactions), CEP250 (10 interactions), TUBGCP2 (6 interactions), MAGED2 (6 interactions) and CEP55 (6 interactions). This revealed two major PCM sub-complexes ( Fig. 1a ), which centre on γ-TuSC and the centriolar protein CEP250 (C-NAP1) [31] . After LGALS3BP antibody validation ( Supplementary Fig. S1 ), we tested a subset of newly identified centrosomal protein-interaction partners for centrosomal localization by antibody and fusion protein overexpression experiments ( Fig. 2 , Supplementary Fig. S2 ). Endogenous LGALS3BP protein is centriole-associated in human osteosarcoma U2OS cells in interphase ( Fig. 2a ) and was detected at lower levels in mitosis with an anti-LGALS3BP antibody. In addition, tagged LGALS3BP showed localization to the interphase centrioles when overexpressed using pre-fixation extraction ( Fig. 2b ). Overexpression without extraction produced a hypertrophic PCM localization as judged by labelling with γ-tubulin as a PCM marker ( Supplementary Fig. S2 ). The localization close to the proximal end of the centrioles (marked by proximity to the procentriole) and to the connecting area between the centrioles ( Fig. 2c ) was independently confirmed by transmission electron microscopy (TEM) pre-embedding and post-embedding immunogold labelling ( Fig. 2d ). This was compared with control IgG labelling to assess labelling specificity ( Fig. 2d ). 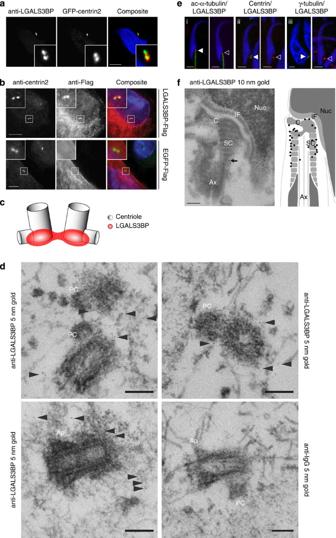Figure 2: LGALS3BP localizes to centrioles. (a) LGALS3BP localizes to the proximal part of centrioles in GFP-centrin-U2OS cells in interphase. The respective labelling with a monoclonal mouse LGALS3BP antibody is shown in red, GFP-centrin in green and 4',6-diamidino-2-phenylindole dihydrochloride (DAPI)-stained DNA in blue in the composite images. Scale bars, 5 μm. (b) Flag-LGALS3BP and Flag-GFP as control were overexpressed in U2OS cells. Flag-LGALS3BP localizes to the centrioles upon pre-fixation extraction and labelling with an anti-Flag antibody (red), an anti-centrin antibody (green) and DAPI-stained DNA (blue). Flag-GFP does not show centriolar labelling. (c) Schematic LGALS3BP localization to the centrioles. (d) TEM immunogold localization of LGALS3BP detected with the mouse LGALS3BP antibody and a 5-nm gold-coupled secondary antibody in U2OS cells. Pre-embedding labelling (top row and bottom right image) and LR-gold post-embedding labelling independently confirmed LGALS3BP localization to the proximal part of centrioles as identified by procentrioles (PC) or presence of the distal centriole subtending appendages (Ap) on the opposite end. The negative control (non-specific IgG antibody) shows no gold labelling. Scale bars, 200 nm. (e) LGALS3BP resides near the proximal part of the distal basal body in rat sperm and testis cryosections. The three panels show single-plane confocal images of earlier and late stage rat sperm labelled with an anti-acetylated α-tubulin antibody (i), anti-centrin antibody (ii) and γ-tubulin antibody (iii) (green), co-labelled with a rabbit anti-LGALS3BP antibody (red). DAPI-stained DNA is shown in blue. Basal body localization of LGALS3BP is detected in earlier stages with centrioles still present (filled arrowheads) and in mature stages after their degeneration (empty arrowheads) as judged by lacking respective markers. (f) Localization of LGALS3BP was confirmed in TEM using pre-embedding labelling with rabbit anti-LGALS3BP and 10 nm gold-coupled secondary antibodies followed by ultrathin sectioning. One to four gold particles were consistently detected at the proximal part of the distal basal body that subtended the flagellar axoneme (Ax) close to the striated columns (SC, arrow). The schematic of the rat sperm head summarizes the observations from a series of images (schematic based on Fawcett, 1975). C, capitulum; IF, implantation fossa; Nuc, Nucleus. Scale bar, 200 nm. Figure 2: LGALS3BP localizes to centrioles. ( a ) LGALS3BP localizes to the proximal part of centrioles in GFP-centrin-U2OS cells in interphase. The respective labelling with a monoclonal mouse LGALS3BP antibody is shown in red, GFP-centrin in green and 4',6-diamidino-2-phenylindole dihydrochloride (DAPI)-stained DNA in blue in the composite images. Scale bars, 5 μm. ( b ) Flag-LGALS3BP and Flag-GFP as control were overexpressed in U2OS cells. Flag-LGALS3BP localizes to the centrioles upon pre-fixation extraction and labelling with an anti-Flag antibody (red), an anti-centrin antibody (green) and DAPI-stained DNA (blue). Flag-GFP does not show centriolar labelling. ( c ) Schematic LGALS3BP localization to the centrioles. ( d ) TEM immunogold localization of LGALS3BP detected with the mouse LGALS3BP antibody and a 5-nm gold-coupled secondary antibody in U2OS cells. Pre-embedding labelling (top row and bottom right image) and LR-gold post-embedding labelling independently confirmed LGALS3BP localization to the proximal part of centrioles as identified by procentrioles (PC) or presence of the distal centriole subtending appendages (Ap) on the opposite end. The negative control (non-specific IgG antibody) shows no gold labelling. Scale bars, 200 nm. ( e ) LGALS3BP resides near the proximal part of the distal basal body in rat sperm and testis cryosections. The three panels show single-plane confocal images of earlier and late stage rat sperm labelled with an anti-acetylated α-tubulin antibody (i), anti-centrin antibody (ii) and γ-tubulin antibody (iii) (green), co-labelled with a rabbit anti-LGALS3BP antibody (red). DAPI-stained DNA is shown in blue. Basal body localization of LGALS3BP is detected in earlier stages with centrioles still present (filled arrowheads) and in mature stages after their degeneration (empty arrowheads) as judged by lacking respective markers. ( f ) Localization of LGALS3BP was confirmed in TEM using pre-embedding labelling with rabbit anti-LGALS3BP and 10 nm gold-coupled secondary antibodies followed by ultrathin sectioning. One to four gold particles were consistently detected at the proximal part of the distal basal body that subtended the flagellar axoneme (Ax) close to the striated columns (SC, arrow). The schematic of the rat sperm head summarizes the observations from a series of images (schematic based on Fawcett, 1975). C, capitulum; IF, implantation fossa; Nuc, Nucleus. Scale bar, 200 nm. Full size image LGALS3BP localization was also identified at the proximal part of the distal basal body in rat spermatozoa whole mounts and in cryosections of rat testis ( Fig. 2e ). Moreover, LGALS3BP continued to remain localized to the basal body region during sperm maturation, even in spermatozoa with a degenerated proximal basal body [32] , [33] ( Fig. 2e ). The distinct localization of LGALS3BP at the proximal part of the basal body in the vicinity of the striated columns in rat sperm was confirmed by pre-embedding labelling in TEM ( Fig. 2f ). Hence, several independent lines of localization experiments confirmed the presence of LGALS3BP at the centriole and in the connecting region between the two parental centrioles. To explore the functional relevance of some of the identified protein interactions revealed by TAP-MS, a subset of nine proteins was selected based on their roles in cancer and other diseases ( Supplementary Data 1 ) and the identification of at least three interactions with known centrosomal proteins. Functional characterization of these proteins via RNAi ( Supplementary Data 2 ) led us to focus our characterization on LGALS3BP. The interaction of LGALS3BP with the γ-TuSC protein TUBG1 was recently reported [34] . LGALS3BP has been described as a secreted extracellular matrix glycoprotein [35] with a role in wound repair in mice [36] . However, neither centrosomal localization nor function has been reported before for LGALS3BP. LGALS3BP depletion affects mitotic spindle and centriole Small interfering RNA (siRNA) depletion of LGALS3BP in U2OS cells resulted in anastral spindle organization ( Fig. 3a ). LGALS3BP depletion also led to free aster-like structures that demonstrated no obvious spatial relationship to the asterless spindle poles ( Fig. 3a ). As the lack of astral microtubules suggested the absence or reduction of centrosome or centriole structure [37] , [38] , we investigated the effect of LGALS3BP depletion (and other identified proteins, Supplementary Fig. S3 , Supplementary Data 2 ) in U2OS cells on centrosome number and structure. Immunofluorescence microscopy showed that LGALS3BP depletion resulted in more than two unequally sized centrosome-like structures ( Fig. 3b ). Multiple centrosome-like structures were also observed in HEK293 cells following LGALS3BP depletion ( Supplementary Fig. S4 ), demonstrating that this phenotype is not restricted to U2OS cells. Subsequently, we investigated whether LGALS3BP (and other identified proteins, Supplementary Fig. S5 ) depletion affected centriole structure or number, which would explain either multiple centrosomes or the lack of aster microtubules. Surprisingly, quantitation of centrioles using an antibody against the centriolar marker centrin [39] revealed an abnormally high percentage of cells with more than two centriole-like structures ( Fig. 4 ). Interestingly, the centriole structures detected were partly not associated with the PCM both in interphase and in mitotic cells ( Fig. 4a ). Fluorescence-activated cell sorting and mitotic index analysis did not reveal an obvious change in cell-cycle distribution or mitotic progression after knockdown ( Supplementary Fig. S6 ). We therefore conclude that a fraction of the present centriole structures is not capable of acquiring PCM and that this feature is not a consequence of cell-cycle dysregulation. To characterize this phenotype further, we determined by immunofluorescence microscopy that the substructures accumulating following LGALS3BP knockdown contained CPAP (a marker found in early stages of centriole assembly), centrin and acetylated tubulin while lacking several other centriolar or centrosomal proteins ( Fig. 4c , Supplementary Fig. S7 , Supplementary Table S1 ), suggesting that LGALS3BP depletion is either required for centriolar assembly or for maintaining centriolar integrity. In addition, to further characterize the phenotype on the ultrastructural level, we conducted TEM of U2OS cells that were transfected with siRNA targeting LGALS3BP or with non-targeting siRNA as control ( Fig. 4d ). TEM revealed, in addition to structurally intact centrioles, an increased presence of centriole-like structures in LGALS3BP-depleted cells ( Fig. 4d ). These structures were represented by incomplete cylinder-like structures and smaller substructures that contained rudimentary microtubule-like structures, also sometimes marked by cytoplasmic microtubules. 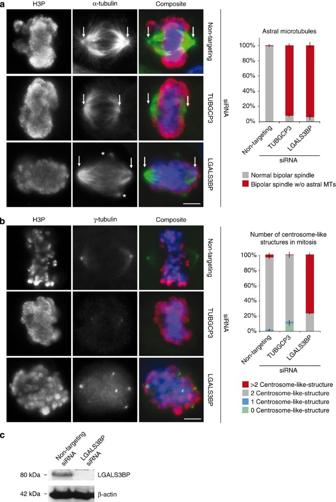Figure 3: Knockdown of LGALS3BP leads to asterless spindle poles and multiple centrosomal structures. (a) LGALS3BP siRNA treatment reveals its function for maintaining astral microtubules in mitotic U2OS cells. Furthermore, LGALS3BP-depleted cells have additional spindle pole-like structures (asterisks) that are detached from the main spindle microtubules. Depletion of positive control TUBGCP3 leads to bipolar asterless spindles. The negative control displays a normal spindle with two poles with aster microtubules after non-targeting siRNA treatment. The respective quantification of presence of astral microtubules is displayed in the chart. Data are shown as means±s.d. of duplicates with an average ofn>90. (b) LGALS3BP depletion leads to supernumerary centrosome-like structures in mitosis, whereas TUBGCP3 siRNA treatment does not affect centrosome-like structure number significantly. The corresponding quantification of the centrosome-like structures is shown in the chart. Data are expressed as means±s.d. of duplicates withn>125 (a,b) Microtubules are labelled with an anti-α-tubulin antibody (green in the composite images ina); centrosome-like structures are labelled with an anti-γ-tubulin antibody (green in the composite images inb). Mitotic chromosomes are labelled with an anti-phosphorylated Histone H3 antibody (red in all composite images). DNA was labelled with DAPI (blue in all composite images). Scale bars, 5 μm. (c) Immunoblotting of U2OS cells treated with LGALS3BP and non-targeting siRNA shows siRNA efficiency and antibody specificity. β-actin was used as loading control. Figure 3: Knockdown of LGALS3BP leads to asterless spindle poles and multiple centrosomal structures. ( a ) LGALS3BP siRNA treatment reveals its function for maintaining astral microtubules in mitotic U2OS cells. Furthermore, LGALS3BP-depleted cells have additional spindle pole-like structures (asterisks) that are detached from the main spindle microtubules. Depletion of positive control TUBGCP3 leads to bipolar asterless spindles. The negative control displays a normal spindle with two poles with aster microtubules after non-targeting siRNA treatment. The respective quantification of presence of astral microtubules is displayed in the chart. Data are shown as means±s.d. of duplicates with an average of n >90. ( b ) LGALS3BP depletion leads to supernumerary centrosome-like structures in mitosis, whereas TUBGCP3 siRNA treatment does not affect centrosome-like structure number significantly. The corresponding quantification of the centrosome-like structures is shown in the chart. Data are expressed as means±s.d. of duplicates with n >125 ( a , b ) Microtubules are labelled with an anti-α-tubulin antibody (green in the composite images in a ); centrosome-like structures are labelled with an anti-γ-tubulin antibody (green in the composite images in b ). Mitotic chromosomes are labelled with an anti-phosphorylated Histone H3 antibody (red in all composite images). DNA was labelled with DAPI (blue in all composite images). Scale bars, 5 μm. ( c ) Immunoblotting of U2OS cells treated with LGALS3BP and non-targeting siRNA shows siRNA efficiency and antibody specificity. β-actin was used as loading control. 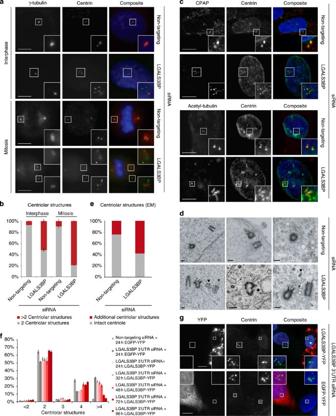Figure 4: Depletion of LGALS3BP leads to supernumerary centriolar structures. (a) siRNA-mediated depletion of LGALS3BP leads to multiple centriolar structures as identified with an anti-centrin antibody both in interphase and in mitotic U2OS cells. There are multiple centrin-positive structures visible that are partly not associated with PCM as marked with an anti-γ-tubulin antibody. The inserts for each image magnify the area of the centrosome. In the composite images, γ-tubulin is displayed in red, centrin in green and DAPI-stained DNA in blue. Scale bars, 5 μm. (b) Quantification of centriolar structures per centrosome. Data are shown as means±s.d. of duplicates withn>200 for each experiment. (c) Centriolar structures resulting from LGALS3BP depletion contain centriolar proteins CPAP and acetylated tubulin in addition to centrin as shown by antibody labelling. CPAP and acetylated tubulin are coloured in red, centrin in green and DAPI-labelled DNA in blue in the composite images. Scale bars, 10 μm. (d) TEM of U2OS cells treated with LGALS3BP siRNAs reveals abnormal centriolar structures indicated by arrowheads. Microtubules emanating from centriolar structures are marked by asterisks. Scale bars, 200 nm. (e) Quantification of centriolar structures determined by TEM withn=37 for non-targeting andn=50 for LGALS3BP siRNA treatment. (f,g) Depletion of endogenous LGALS3BP using a siRNA pool targeting the 3′ untranslated region (3′UTR) of LGALS3BP with simultaneous overexpression of exogenous LGALS3BP-YFP up to 96 h decreases the supernumerary centriolar structures up to control ranges in U2OS cells (immunoblotting inSupplementary Fig. S1). (f) Quantification of the centriolar structures in the LGALS3BP-rescue experiment. Data are expressed as means±s.d. of triplicates with eachn>200. (g) Cells depleted for endogenous LGALS3BP show normal centriole number when LGALS3BP-YFP is expressed demonstrating the rescue of centriolar LGALS3BP-depletion phenotypes. This is not the case in cells expressing EGFP-YFP as control. The composite images show LGALS3BP-YFP and EGFP-YFP in red, centrin in green and DAPI-labelled DNA in blue. The asterisk indicates a LGALS3BP-YFP-transfected cell with rescue adjacent to an untransfected cell with supernumerary centriolar structures. Scale bars, 10 μm. Full size image Figure 4: Depletion of LGALS3BP leads to supernumerary centriolar structures. ( a ) siRNA-mediated depletion of LGALS3BP leads to multiple centriolar structures as identified with an anti-centrin antibody both in interphase and in mitotic U2OS cells. There are multiple centrin-positive structures visible that are partly not associated with PCM as marked with an anti-γ-tubulin antibody. The inserts for each image magnify the area of the centrosome. In the composite images, γ-tubulin is displayed in red, centrin in green and DAPI-stained DNA in blue. Scale bars, 5 μm. ( b ) Quantification of centriolar structures per centrosome. Data are shown as means±s.d. of duplicates with n >200 for each experiment. ( c ) Centriolar structures resulting from LGALS3BP depletion contain centriolar proteins CPAP and acetylated tubulin in addition to centrin as shown by antibody labelling. CPAP and acetylated tubulin are coloured in red, centrin in green and DAPI-labelled DNA in blue in the composite images. Scale bars, 10 μm. ( d ) TEM of U2OS cells treated with LGALS3BP siRNAs reveals abnormal centriolar structures indicated by arrowheads. Microtubules emanating from centriolar structures are marked by asterisks. Scale bars, 200 nm. ( e ) Quantification of centriolar structures determined by TEM with n =37 for non-targeting and n =50 for LGALS3BP siRNA treatment. ( f , g ) Depletion of endogenous LGALS3BP using a siRNA pool targeting the 3′ untranslated region (3′UTR) of LGALS3BP with simultaneous overexpression of exogenous LGALS3BP-YFP up to 96 h decreases the supernumerary centriolar structures up to control ranges in U2OS cells (immunoblotting in Supplementary Fig. S1 ). ( f ) Quantification of the centriolar structures in the LGALS3BP-rescue experiment. Data are expressed as means±s.d. of triplicates with each n >200. ( g ) Cells depleted for endogenous LGALS3BP show normal centriole number when LGALS3BP-YFP is expressed demonstrating the rescue of centriolar LGALS3BP-depletion phenotypes. This is not the case in cells expressing EGFP-YFP as control. The composite images show LGALS3BP-YFP and EGFP-YFP in red, centrin in green and DAPI-labelled DNA in blue. The asterisk indicates a LGALS3BP-YFP-transfected cell with rescue adjacent to an untransfected cell with supernumerary centriolar structures. Scale bars, 10 μm. Full size image The centriolar substructure-accumulation phenotype could be rescued by overexpression of yellow fluorescent protein (YFP)-tagged LGALS3BP while specifically depleting endogenous protein using 3′ untranslated region (3′UTR) targeting siRNAs ( Fig. 4f ). The efficiency of the siRNAs used to independently confirm the LGALS3BP phenotype is shown in Supplementary Fig. S1 (for sequences see Supplementary Data 2 ). To better understand the origin of the centriolar substructures, we analysed the distribution of mature centriole marker glutamylated tubulin [40] and daughter centriole marker CNTROB. Quantification of these markers after LGALS3BP knockdown ( Fig. 5 ) revealed that the number of both parental and daughter centrioles is maintained, whereas the number of centrin-containing centriolar substructures is increasing several fold ( Fig. 5b ), suggesting that those structures are not likely to be derived from parental or daughter centrioles or do not block their assembly. 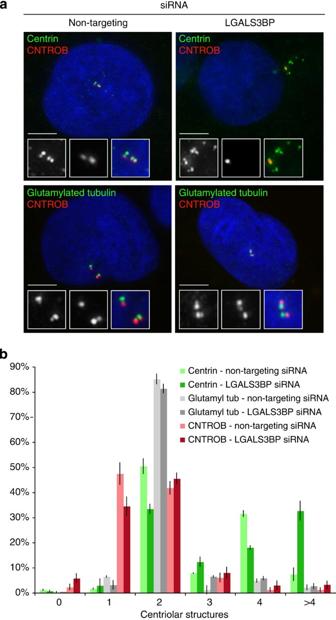Figure 5: Centriolar structures after LGALS3BP siRNA lack parental and daughter centriole markers. To characterize the supernumerary centriolar structures that are observed following LGALS3BP depletion, the presence of markers for daughter centrioles (CNTROB) and parental centrioles (glutamylated tubulin) on those structures in comparison with centrin was quantified. (a) Immunofluorescence microscopy analysis of U2OS cells treated with siRNA against LGALS3BP revealed that the number of both parental and daughter centrioles stays constant, whereas the number of centrin-positive structures increases. Magnifications of the centrioles are shown in the inserts on the bottom of each image. Nuclei are labelled with DAPI. Scale bars, 5 μm. (b) The quantification of centriolar structures as labelled with antibodies against glutamylated tubulin, CNTROB and centrin reflects that daughter centrioles and parental centrioles are not affected by LGALS3BP knockdown. The data are expressed as means±s.d. of duplicates with eachn>200. Figure 5: Centriolar structures after LGALS3BP siRNA lack parental and daughter centriole markers. To characterize the supernumerary centriolar structures that are observed following LGALS3BP depletion, the presence of markers for daughter centrioles (CNTROB) and parental centrioles (glutamylated tubulin) on those structures in comparison with centrin was quantified. ( a ) Immunofluorescence microscopy analysis of U2OS cells treated with siRNA against LGALS3BP revealed that the number of both parental and daughter centrioles stays constant, whereas the number of centrin-positive structures increases. Magnifications of the centrioles are shown in the inserts on the bottom of each image. Nuclei are labelled with DAPI. Scale bars, 5 μm. ( b ) The quantification of centriolar structures as labelled with antibodies against glutamylated tubulin, CNTROB and centrin reflects that daughter centrioles and parental centrioles are not affected by LGALS3BP knockdown. The data are expressed as means±s.d. of duplicates with each n >200. Full size image Furthermore, the generation of centriolar substructures upon LGALS3BP depletion was found to depend on the presence of the centriole-duplication factor PLK4 as co-depletion of PLK4 and LGALS3BP reduced the number of generated centriolar structures from 60% (LGALS3BP siRNA) to 20% (PLK4 and LGALS3BP siRNA) as opposed to 8% for control cells (PLK4 siRNA and non-targeting control siRNA) ( Fig. 6a ). As a large fraction of cells (75–85%) retains at least one centriole, both in the case of the PLK4 knockdown and the simultaneous knockdown of PLK4 and LGALS3BP, it is likely that the observed decrease of cells with supernumerary centriolar structures can be explained by a dependence of this phenotype on PLK4 rather than a lack of centrioles caused by abrogation of centriole duplication through PLK4 depletion. 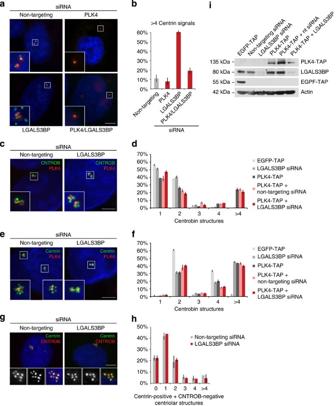Figure 6: The formation of centriole-like structures after LGALS3BP depletion depends on PLK4. (a,b) Immunofluorescence microscopy and quantification of supernumerary centriole-like structures in U2OS cells after siRNA depletion of LGALS3BP and PLK4, as well as simultaneous depletion of both proteins. Knockdown of PLK4 in LGALS3BP-depletion background reveals a significant decrease of cells with >4 centrin-positive signals. (a) Immunofluorescence microscopy was conducted using antibodies against γ-tubulin and centrin. In the composite image γ-tubulin is shown in red, centrin in green and DAPI-stained DNA in blue. Scale bar, 5 μm for all images. (b) Data are expressed as means±s.d. of duplicates withn>200. (c–f) Immunofluorescence microscopy and quantification of supernumerary daughter centriolar marker CNTROB (c,d) and centrin (e,f) in U2OS cells after transient PLK4-TAP overexpression in the background of LGALS3BP depletion shows no difference in the formation of multiple procentrioles compared with non-targeting siRNA background and relevant controls. (c,e) PLK4-TAP was labelled with rabbit IgG shown in red, antibody-labelled CNTROB or centrin in green and DAPI-stained DNA in blue. Scale bars, 5 μm. (d,f) Data are expressed as means±s.d. of triplicates withn>200. (g) Immunofluorescence microscopy of stable myc-PLK4-U2OS cells after 24 h tetracycline induction in the background of LGALS3BP depletion shows no significant difference in number and localization of centrin and CNTROB compared with the background of non-targeting siRNA treatment. In the composite images, the labelling with specific antibodies is shown in green for centrin and in red for CNTROB. DAPI-stained DNA is shown in blue. The inserts at the bottom magnify the area of the centrioles. Scale bar, 5 μm. (h) The quantification of centriolar structures that are centrin-positive but centrobin-negative reveals no significant change after myc-PLK4 induction in a LGALS3BP-depletion background compared with the background of non-targeting siRNA treatment. Data are expressed as means±s.d. of duplicates withn>200. (i) Verification of the experiments inc–fby immunoblotting. Exogenous EGFP-TAP and PLK4-TAP is detected with rabbit IgG and LGALS3BP with a specific rabbit antibody. β-actin was used as loading control. Figure 6: The formation of centriole-like structures after LGALS3BP depletion depends on PLK4. ( a , b ) Immunofluorescence microscopy and quantification of supernumerary centriole-like structures in U2OS cells after siRNA depletion of LGALS3BP and PLK4, as well as simultaneous depletion of both proteins. Knockdown of PLK4 in LGALS3BP-depletion background reveals a significant decrease of cells with >4 centrin-positive signals. ( a ) Immunofluorescence microscopy was conducted using antibodies against γ-tubulin and centrin. In the composite image γ-tubulin is shown in red, centrin in green and DAPI-stained DNA in blue. Scale bar, 5 μm for all images. ( b ) Data are expressed as means±s.d. of duplicates with n >200. ( c – f ) Immunofluorescence microscopy and quantification of supernumerary daughter centriolar marker CNTROB ( c , d ) and centrin ( e , f ) in U2OS cells after transient PLK4-TAP overexpression in the background of LGALS3BP depletion shows no difference in the formation of multiple procentrioles compared with non-targeting siRNA background and relevant controls. ( c , e ) PLK4-TAP was labelled with rabbit IgG shown in red, antibody-labelled CNTROB or centrin in green and DAPI-stained DNA in blue. Scale bars, 5 μm. ( d , f ) Data are expressed as means±s.d. of triplicates with n >200. ( g ) Immunofluorescence microscopy of stable myc-PLK4-U2OS cells after 24 h tetracycline induction in the background of LGALS3BP depletion shows no significant difference in number and localization of centrin and CNTROB compared with the background of non-targeting siRNA treatment. In the composite images, the labelling with specific antibodies is shown in green for centrin and in red for CNTROB. DAPI-stained DNA is shown in blue. The inserts at the bottom magnify the area of the centrioles. Scale bar, 5 μm. ( h ) The quantification of centriolar structures that are centrin-positive but centrobin-negative reveals no significant change after myc-PLK4 induction in a LGALS3BP-depletion background compared with the background of non-targeting siRNA treatment. Data are expressed as means±s.d. of duplicates with n >200. ( i ) Verification of the experiments in c – f by immunoblotting. Exogenous EGFP-TAP and PLK4-TAP is detected with rabbit IgG and LGALS3BP with a specific rabbit antibody. β-actin was used as loading control. Full size image We asked the question if the number of centriole structures increases when centriole duplication is induced by overexpression of PLK4 in the background of LGALS3BP knockdown. Surprisingly, we did not see an increase in supernumerary centriole structures ( Fig. 6c–f ) under these conditions. To discriminate an increase of centriolar structures generated through LGALS3BP depletion from the PLK4 overexpression effect, we utilized stable PLK4-overexpressing U2OS cells [40] to quantify centriolar structures following LGALS3BP depletion that comprise centrin, but not CNTROB ( Fig. 6g ). As supernumerary centriolar structures contained both proteins, we conclude that PLK4 overexpression compensates LGALS3BP depletion. Collectively, our results indicate that LGALS3BP is suppressing the generation of supernumerary centriolar substructures under the control of PLK4. To further explore the molecular role of LGALS3BP concerning the centrosome, we investigated the effect of overexpression on the centrosome. Overexpression of LGALS3BP leads to PCM hypertrophy Overexpression of LGALS3BP in HEK293 cells was found to lead to PCM dispersion showing diffuse γ-tubulin localization over an enlarged PCM area ( Supplementary Figs S4 and S8 ) resembling typical centrosome abnormalities frequently detected in high-grade cancer tissues [22] . To explore the molecular basis of the observed PCM abnormalities, we analysed the function of the predicted LGALS3BP domains. The LGALS3BP sequence can be divided into six stretches [41] with four predicted functional/structural domains: the signal sequence domain (1–18) is a putative unconventional secretion leader sequence, followed by a surface ligand-binding domain (SRCR domain 1; scavenger receptor Cys-rich domain; 19–133), the BTB/POZ domain (domain 2; 127–251; BTB for BR-C, ttk and bab; POZ for Pox virus and Zinc finger), the intervening region (IVR; domain 3; 251–407), a linker sequence (408–451) and domain 4 (452–585) with no particular homology to other proteins. Overexpression of different deletion constructs ( Supplementary Fig. S8 ) revealed that expression of the IVR domain is required for the PCM dispersion. This domain together with the BTB/POZ region is (partly) homologous to a kelch protein [41] that facilitates oligomerization, suggesting that protein oligomerization might be critical for PCM dispersion caused by LGALS3BP overexpression. In addition, our results demonstrated that the signal sequence is not required for PCM dispersion, implying that secretion of LGALS3BP is not causally linked to the observed centrosome dispersion. This is consistent with the result that neither overexpression nor depletion of LGALS3, which has been suggested to bind to LGALS3BP on the cell surface [42] , was found to display a centrosome- or spindle-related phenotype ( Supplementary Fig. S9 ) in U2OS and HEK293 cells, respectively. This argues for a centrosome-related role of the intracellular LGALS3BP in human somatic cells. Dysregulated LGALS3BP correlates with abnormal centrosomes To determine whether the LGALS3BP overexpression phenotype is also detected when native LGALS3BP protein is endogenously upregulated, we selected the breast cancer cell line SK-BR-3 because it shows one of the highest LGALS3BP expressions among a large number of different cancer cell lines with elevated protein levels of LGALS3BP ( http://www.proteinatlas.org ) and compared it with the MCF10A non-tumorigenic mammary epithelial cell line that expresses LGALS3BP at normal levels ( Fig. 7a ). 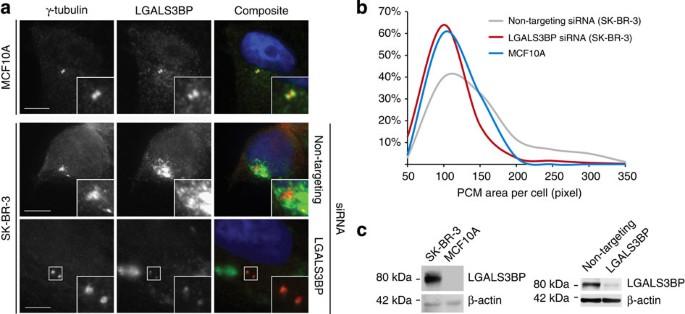Figure 7: LGALS3BP knockdown rescues PCM dispersion in LGALS3BP endogenously overexpressing cells. (a) LGALS3BP is highly expressed in the breast cancer cell line SK-BR-3 as compared with non-tumorigenic breast epithelial cell line MCF10A. Centrosomes are hypertrophic in SK-BR-3 cells, whereas centrosome morphology in MCF10A cells is normal. The siRNA depletion of LGALS3BP in SK-BR-3 cells reverts the centrosome dispersion phenotype, resembling normal centrosomes as in MCF10A cells. After pre-fixation extraction, the cells were labelled for PCM with an anti-γ-tubulin antibody shown in red in the composite image, LGALS3BP was labelled with a mouse antibody shown in green and DNA was stained with DAPI shown in blue in the composite image. Scale bars, 5 μm. (b) PCM hypertrophy of SK-BR-3 cells as opposed to normal centrosomes of MCF10A cells was quantified using an image analysis macro in ImageJ that determines the total area of PCM per cell. The diagram shows a comparison of the PCM area of MCF10A cells, SK-BR-3 cells and LGALS3BP-depleted SK-BR-3 cells, visualizing the decrease of PCM area and therefore a rescue of the PCM hypertrophy phenotype. The cells were tested in triplicates with eachn>200. The percentage of cells that has been assigned to an interval of pixel numbers describing the area of the PCM for each cell type or knockdown including s.d. can be found inSupplementary Table S1. (c) Immunoblotting with a rabbit anti-LGALS3BP antibody shows that the SK-BR-3 cell line has a highly elevated level of LGALS3BP, whereas the MCF10A cell line has normal level of LGALS3BP (left panel). The endogenous level of LGALS3BP in MCF10A cells cannot be displayed to avoid complete overexposure of the blot through the SK-BR-3 sample. Therefore, exposure is only shown close to signal saturation for the SK-BR-3 cells. The right panel shows reduction of the endogenous LGALS3BP levels in SK-BR-3 cells after siRNA treatment corresponding to the experiments shown inb. β-actin (both panels) was used as a loading control. Figure 7: LGALS3BP knockdown rescues PCM dispersion in LGALS3BP endogenously overexpressing cells. ( a ) LGALS3BP is highly expressed in the breast cancer cell line SK-BR-3 as compared with non-tumorigenic breast epithelial cell line MCF10A. Centrosomes are hypertrophic in SK-BR-3 cells, whereas centrosome morphology in MCF10A cells is normal. The siRNA depletion of LGALS3BP in SK-BR-3 cells reverts the centrosome dispersion phenotype, resembling normal centrosomes as in MCF10A cells. After pre-fixation extraction, the cells were labelled for PCM with an anti-γ-tubulin antibody shown in red in the composite image, LGALS3BP was labelled with a mouse antibody shown in green and DNA was stained with DAPI shown in blue in the composite image. Scale bars, 5 μm. ( b ) PCM hypertrophy of SK-BR-3 cells as opposed to normal centrosomes of MCF10A cells was quantified using an image analysis macro in ImageJ that determines the total area of PCM per cell. The diagram shows a comparison of the PCM area of MCF10A cells, SK-BR-3 cells and LGALS3BP-depleted SK-BR-3 cells, visualizing the decrease of PCM area and therefore a rescue of the PCM hypertrophy phenotype. The cells were tested in triplicates with each n >200. The percentage of cells that has been assigned to an interval of pixel numbers describing the area of the PCM for each cell type or knockdown including s.d. can be found in Supplementary Table S1 . ( c ) Immunoblotting with a rabbit anti-LGALS3BP antibody shows that the SK-BR-3 cell line has a highly elevated level of LGALS3BP, whereas the MCF10A cell line has normal level of LGALS3BP (left panel). The endogenous level of LGALS3BP in MCF10A cells cannot be displayed to avoid complete overexposure of the blot through the SK-BR-3 sample. Therefore, exposure is only shown close to signal saturation for the SK-BR-3 cells. The right panel shows reduction of the endogenous LGALS3BP levels in SK-BR-3 cells after siRNA treatment corresponding to the experiments shown in b . β-actin (both panels) was used as a loading control. Full size image Comparison of centrosome morphology in these cell lines revealed tightly focused centrosomes in MCF10A cells, whereas SK-BR-3 cells had centrosomes with a diffuse appearance and increased PCM area ( Fig. 7a ) as determined by pixel-based quantification of centrosome size ( Fig. 7b , Supplementary Table S2 ). Hence, the morphology of the centrosomes in SK-BR-3 cells strongly resembles the CMV promoter-driven LGALS3BP-overexpression phenotype in HEK293 cells ( Supplementary Fig. S8 ). To test whether endogenous LGALS3BP overexpression is functionally linked to centrosome hypertrophy, we conducted siRNA-mediated depletion in SK-BR-3 cells. Reduction of LGALS3BP protein levels ( Fig. 7c ) in the endogenous LGALS3BP-upregulated cells resulted in a decrease of the percentage of cells with a larger PCM area and therefore rescued the normal centrosome phenotype ( Fig. 7a ). LGALS3BP is frequently dysregulated in cancer tissue [43] , [44] . In view of this and our findings in cells, we investigated whether patients’ tissues with dysregulated levels of LGALS3BP expression also exhibit centrosome and centriole abnormalities in situ . We screened an array of the 17 most common human tumours (total 209 samples, Supplementary Data 3 ) by RT–PCR to identify tissue samples that showed a large discrepancy of LGALS3BP mRNA levels between cancer and control tissues ( Fig. 8a ). We measured abnormally low expression levels of both mRNA (eight-fold downregulation in tumour) and protein ( Fig. 8b ) in seminoma tissue showing typical tumour nodules ( Fig. 8c ). Immunofluorescence microscopy of corresponding sections from the same tissues detected abnormal PCM and accumulation of centriole-like structures ( Fig. 8d ) that closely phenocopied the results of LGALS3BP siRNA experiments in U2OS cells ( Fig. 4 ). In addition, abnormally shaped centrosomes were associated with aberrant chromosomal configurations ( Fig. 8d ). In cryosections of the normal control testis tissue, mitotic cells were rare and no such abnormalities could be detected. 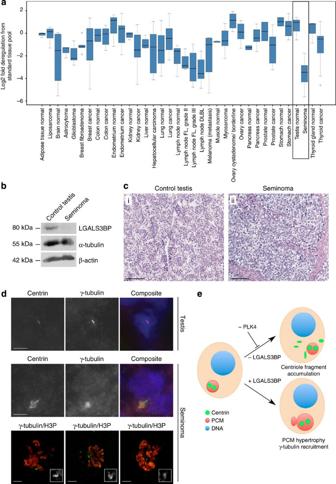Figure 8: Centrosome aberrations are detected in seminoma tissue with abnormally low LGALS3BP levels. (a) RT–PCR quantification of different human tumour tissues was used to identify tissues with deregulated LGALS3BP levels when compared with relevant control tissue. The strongest deregulation is present in testis, where the expression of LGALS3BP is eight-fold downregulated in the seminoma (boxed). Immunoblotting, haematoxylin staining analysis and immunofluorescence microscopy for corresponding tissue samples are shown inb–d. (b) Immunoblotting of the control testis tissue shows normal LGALS3BP protein levels, which are abnormally reduced in seminoma cancer tissue. α-tubulin and β-actin were used as loading controls. (c) Haematoxylin-stained cryosection of testis (i) and seminoma (ii) tissue. Seminoma with sheet-like arrangement of cells with clear cytoplasm, well-defined cell membranes, and nuclei with prominent, central nucleoli. Tumour nodules are subdivided by branching, fibrous septa containing few lymphocytes. Normal testis with clusters of Leydig cells. Seminiferous tubules are lined by Sertoli cells. Occasional representation of spermatogenesis. Scale bars, 200 μm. (d) Cryosections of human testis control tissue (first row) and human seminoma tissue (second row). The control tissue shows both normal-sized centrioles and PCM, whereas in the seminoma aberrant, centriolar structures are detected with and without associated PCM. In the composite images, anti-centrin labelling is shown in green, γ-tubulin in red and DAPI-stained DNA in blue. Scale bars, 5 μm. In the third row, confocal microscopy image projections of double-labelled mitotic cells in seminoma tissue with phosphorylated Histone H3 (red) and γ-tubulin (green) are shown. Inserts on the bottom of each image show an enlarged view of the centrosome. Abnormally distributed chromosomes are frequently detected in cells correlating with aberrant shaped centrosomes. (e) Model describing the interrelation between deregulation of LGALS3BP and PLK4-dependent centriolar structure accumulation and PCM hypertrophy, respectively. Figure 8: Centrosome aberrations are detected in seminoma tissue with abnormally low LGALS3BP levels. ( a ) RT–PCR quantification of different human tumour tissues was used to identify tissues with deregulated LGALS3BP levels when compared with relevant control tissue. The strongest deregulation is present in testis, where the expression of LGALS3BP is eight-fold downregulated in the seminoma (boxed). Immunoblotting, haematoxylin staining analysis and immunofluorescence microscopy for corresponding tissue samples are shown in b – d . ( b ) Immunoblotting of the control testis tissue shows normal LGALS3BP protein levels, which are abnormally reduced in seminoma cancer tissue. α-tubulin and β-actin were used as loading controls. ( c ) Haematoxylin-stained cryosection of testis (i) and seminoma (ii) tissue. Seminoma with sheet-like arrangement of cells with clear cytoplasm, well-defined cell membranes, and nuclei with prominent, central nucleoli. Tumour nodules are subdivided by branching, fibrous septa containing few lymphocytes. Normal testis with clusters of Leydig cells. Seminiferous tubules are lined by Sertoli cells. Occasional representation of spermatogenesis. Scale bars, 200 μm. ( d ) Cryosections of human testis control tissue (first row) and human seminoma tissue (second row). The control tissue shows both normal-sized centrioles and PCM, whereas in the seminoma aberrant, centriolar structures are detected with and without associated PCM. In the composite images, anti-centrin labelling is shown in green, γ-tubulin in red and DAPI-stained DNA in blue. Scale bars, 5 μm. In the third row, confocal microscopy image projections of double-labelled mitotic cells in seminoma tissue with phosphorylated Histone H3 (red) and γ-tubulin (green) are shown. Inserts on the bottom of each image show an enlarged view of the centrosome. Abnormally distributed chromosomes are frequently detected in cells correlating with aberrant shaped centrosomes. ( e ) Model describing the interrelation between deregulation of LGALS3BP and PLK4-dependent centriolar structure accumulation and PCM hypertrophy, respectively. Full size image The interaction network described here identifies new protein–protein interactions that can now be further exploited to define functional modules and components that mediate protein–protein interactions in the centrosome or modulate centrosomal protein functions. We show a particular example of such a molecule, namely LGALS3BP, a centriole-associated protein that functions in controlling centriole biogenesis. In addition, LGALS3BP levels are critical for overall centrosome structure and function as increase or decrease of its protein levels leads to PCM dispersion and defective microtubule aster formation, respectively. Furthermore, LGALS3BP-interacting protein CEP55 is a molecular hub that is associated with CEP76, Aurora A, VCP, TUBGCP3 and p53, suggesting that CEP55 has a critical role in the regulation of centrosome function or structure. A role for CEP55 in cytokinesis has previously been suggested [45] . MAGED2, a p53 dissociator in yeast [46] is linked to TUBGCP3, CEP250 and p53. This extends and further corroborates the association of molecules of the p53 signalling pathway with the centrosome [27] . The network provides new information on protein–protein interactions and suggests potential regulatory dependencies for the mitotic kinase Aurora A as both CEP192 and CEP55 interact with this kinase. The interaction network also predicts additional new centrosomal components. We suggest that such candidates that have been identified to interact with multiple different centrosomal proteins are likely to be transiently or stably associated with the centrosome, though they remain to be confirmed as centrosomal in the future. Centrosome abnormalities in morphology and number are a hallmark of advanced cancer [22] , [26] and several causative molecular mechanisms for these aberrations, for example, dysregulation of cell-cycle regulatory proteins, checkpoint components and related pathways through gene mutation, gene amplification or the introduction of viral factors through infection [27] , [47] have been proposed. However, the molecular basis of such mechanisms of centrosome abnormalities and their link to the cancer regulatory pathways remains to be elucidated in detail. Our approach identified and characterized known and previously unknown centrosomal protein components and analysed their relevance concerning centrosome aberrations in cancer. In proliferating somatic human cells, controlled LGALS3BP protein levels are required for centriole biogenesis and are essential for the structural cohesion of the PCM and spindle organization. We demonstrated in HEK293 cells that the LGALS3BP IVR domain that facilitates LGALS3BP oligomerization [41] is critical for induction of PCM hypertrophy. This effect of LGALS3BP dysregulation was reflected in human cancer cells (SK-BR-3, high levels of LGALS3BP protein) and human seminoma cancer tissue (low levels of LGALS3BP protein and mRNA). The fact that we could reverse the centrosome hypertrophy phenotype in SK-BR-3 cells by depletion of endogenously overexpressed LGALS3BP suggests that dysregulation of LGALS3BP might indeed contribute to the centrosome abnormalities observed in high-grade cancer cells. In cells with phenotypically normal centrosomes, the effect of LGALS3BP depletion is distinct from the functional inhibition of other major centrosome proteins, for example, the γ-TuSC components TUBGCP3, TUBGCP2, PCNT and PCM-1 [48] , [49] that lead to PCM depletion and/or monopolar spindles. In contrast, LGALS3BP depletion leads to accumulation of centriolar substructures that often lack PCM, which resembles the RNAi phenotype of the centriolar component NME7 ( Supplementary Fig. S5 ) and centriolin, a component of the subdistal appendages of the mature centriole [48] , [50] . The accumulation of centriolar substructures upon LGALS3BP depletion, the protein–protein interactions with the centrosomal core proteins of the γ-TuSC and with the centriolar protein CEP250 plus the close centriolar association in somatic cells, as well as sperm basal body association, all strongly argue for LGALS3BP to be a centriolar protein. However, an indirect effect of the depletion of a PCM component on centriole assembly cannot be excluded as this effect has also been suggested before for some PCM proteins [51] . The observed phenotypes resulting from overexpression or depletion in cultured cells, as well as endogenous up- or downregulation of LGALS3BP in cancer cells, are summarized in the proposed model ( Fig. 8e ). A low level of the protein leads to the accumulation of centriolar structures, comprising acetylated tubulin, CPAP and centrin frequently not being associated with PCM. In contrast, PCM hypertrophy is likely to be caused through increased γ-tubulin recruitment as a consequence of a high LGALS3BP level that might sequester TUBGCP3 and other PCM components to the centrosome. The fact that co-depletion of LGALS3BP and PLK4 leads to less frequent occurrence of the LGALS3BP accumulation of centriolar structure-phenotype suggests that PLK4 depletion is the rate limiting step for centriole duplication, and hence less centriolar structures are produced when simultaneously depleting LGALS3BP. This is consistent with the fact that the number of parental centrosomes and daughter centrioles is maintained after LGALS3BP depletion, suggesting that the observed centriolar substructures are not likely to originate from disassembly of parental and daughter centrioles. In addition, LGALS3BP downregulation in the background of PLK4 overexpression shows no obvious increase in centriole-like structures. This suggests that PLK4 overwrites the effect of LGALS3BP depletion, which we propose could be the repression of the accumulation of centriolar complexes. We could not detect an effect of LGALS3BP depletion on the PLK4-driven procentriole assembly in this type of experiments [40] . Formally, we cannot exclude that the generated structures are the result from disintegrating procentriolar structures. However, we regard this as unlikely as we could not detect CNTROB, SAS6 and CEP135 on these structures. Our results suggest, supported by our interaction and functional data, that LGALS3BP is a centriolar component that is functioning as a break for centriolar assembly. However, as we did not detect other markers of early centriolar assembly, namely PLK4, SAS6 and CEP135, we think that the identified structures do not represent typical early events but rather intermediate steps of centriolar assembly. Recently, LGALS3—an extracellular signalling molecule and interacting partner of LGALS3BP—was shown to be transiently associated with the centrosome in postconfluent MDCK cells. In LGALS3-knockout mice and in postconfluent MDCK cells depleted of LGALS3 by siRNA, centrosome defects and supernumerary centrin-positive structures were observed [52] . Hence, the suggested role of LGALS3 in epithelial morphogenesis [52] argues for a critical developmental role for this binding protein that is not detected in proliferating somatic cells by overexpression and depletion experiments. Taken these results together with our experiments that deplete LGALS3 from proliferating U2OS cells without resulting in significant effects on centrosome or centriole number is consistent with a centrosome-related phenotype of LGALS3 in differentiated or postconfluent cells. We discovered a striking endogenous localization of LGALS3BP at the proximal part of the distal basal body in rat sperm. Surprisingly, the localization was even maintained in spermatozoa, in which no proximal centriole could be detected and γ-tubulin and centrin staining were absent. In this context, the fact that maturing rat spermatozoa are losing their proximal centriole and degenerating their distal centriole [32] , [33] suggests that LGALS3BP is part of a proximal structure of the basal body that connects the centriole to the capitulum [53] in the sperm head. This is consistent with the immunogold localization experiments we have carried out for LGALS3BP in U2OS cells and the protein–protein interaction we identified for LGALS3BP with CEP250 ( Fig. 1a ) that is localized to the proximal end of the centriole [31] . The localization of LGALS3BP in sperm basal bodies and centrioles in somatic cells and its critical role in centriole biogenesis in proliferating somatic cells suggest an important role in a wide variety of tissues, developmental stages and in diseases. Taken together our results suggest that some of the centrosomal/centriolar abnormalities in cancer are likely to be based on the accumulation of centriole structures by deregulation of centriolar components, hence providing another possible link between centrosome dysfunction and tumorigenesis [54] . Tandem affinity purification TAP was performed from total lysates of either transient transfected 293-F cells or stably transfected HEK293 Flp-In TRex cells as described previously [55] . Cell pellets were resuspended in lysis buffer (10%(w/v) glycerol, 50 mM Hepes-KOH pH 8.0, 100 mM KCl, 2 mM EDTA, 0.1%(w/v) NP-40, 2 mM dithiothreitol, 1 × protease inhibitor mix, 10 mM NaF, 0.25 mM NaOVO 3 , 5 nM okadaic acid, 5 nM calyculin A and 50 mM β-glycerophosphate) and incubated for 30 min on ice followed by two freeze-thaw cycles. After centrifugation, the supernatant was kept. The following steps were carried out at 4 °C with pre-chilled buffers, and washing steps were performed three times with 10 volumes of the corresponding buffer. IgG Sepharose 6 Fast Flow beads (Amersham Biosciences) were washed with lysis buffer and incubated with cell lysates under rotation for 4 h. Spun-down IgG beads were washed with lysis buffer and then with TEV buffer (10 mM Hepes-KOH pH 8.0, 150 mM NaCl, 0.1%(w/v) NP-40, 500 μM EDTA, 1 mM dithiothreitol and 1 × protease inhibitor). IgG beads were resuspended in TEV buffer containing the TEV protease (purified by our laboratory, plasmid kindly provided by B Séraphin) and incubated mixing overnight. Calmodulin Sepharose 4B beads (Amersham Biosciences) were washed with calmodulin-binding buffer (10 mM β-mercaptoethanol, 10 mM Hepes-KOH pH 8.0, 150 mM NaCl, 1 mM Mg(OAc) 2 , 1 mM imidazole, 0.1%(w/v) NP-40 and 2 mM CaCl 2 ). IgG beads were eluted and washed with calmodulin-binding buffer using Handee centrifuge columns (Pierce). After centrifugation, the flow-through was mixed with 1/250 volume 1 M CaCl 2 and incubated with the calmodulin beads for 2 h. Spun-down calmodulin beads were washed with calmodulin-binding buffer and subsequently with calmodulin-rinsing buffer (50 mM ammonium bicarbonate pH 8.0, 75 mM NaCl, 1 mM Mg(OAc) 2 , 1 mM imidazole and 2 mM CaCl 2 ). Calmodulin beads were transferred to a new Handee centrifuge column, resuspended with calmodulin-elution buffer (50 mM ammonium bicarbonate pH 8.0 and 25 mM EGTA) and incubated 20 min under rotation. Proteins were eluted twice by centrifugation and then analysed by SDS–PAGE, immunoblotting and MS. We defined a false-positive list from our negative TAP controls: non-transfected cells, green fluorescent protein (GFP) as bait protein and IgG beads control ( Supplementary Data 1 ). Immunoprecipitation Protein-G magnetic beads (Dynal) were cross-linked with a mouse monoclonal anti-myc (Upstate), anti-flag (Sigma) or anti-GFP (Roche) antibody and with non-immune rabbit IgG (Jackson ImmunoResearch) following the manufacturer’s instructions. Cells were lysed in buffer containing 10%(w/v) glycerol, 0.5%(w/v) NP-40, 20 mM Hepes, 0.1 M NaCl, 2 mM EGTA, 2 mM β-mercaptoethanol, 2 mM PMSF, 2 mM Na 3 VO 4 , 1 mM NaF, 25 mM β-glycerophosphate and protease inhibitors. Protein extracts were pre-incubated with protein-G magnetic beads for 30 min at 4 °C. The beads were removed and the cleared extracts were incubated with anti-myc, anti-flag or anti-GFP and IgG-coated beads for 4 h at 4 °C. After washing the beads, the bound protein complexes were eluted for 30 min at 4 °C on a thermomixer using RapiGest SF Surfactant (Waters Corporation) as a 0.1% solution in elution buffer containing 20 mM Hepes, 0.1 M NaCl, 2 mM EGTA and 2 mM β-mercaptoethanol. Isolated complexes were analysed by SDS–PAGE, immunoblotting or MS. RNA interference Knockdown was performed in HEK293, SK-BR-3 or U2OS cells. The siRNA oligonucleotides were obtained from Dharmacon. Transfection of siRNAs was performed with DharmaFect1 (Dharmacon) according to the manufacturer’s instructions. The day before siRNA transfection, 90,000–300,000 cells were seeded per well of a six-well plate. Analysis was performed 72 h after transfection. Tissue cryosections and tissue preparation Human tumour ( n ~10) and normal ( n ~3) tissue samples of the main organs (adipose tissue, brain, breast, colon, endometrium, kidney, liver, lung, lymphatic system, muscle, ovary, pancreas, prostate, stomach, testis and thyroid gland) were collected from the Tissue Bank of the Medical University of Graz. Approval by the Ethical Committee of the Medical University of Graz (EK 20-404 ex 08/09) and informed consent of the donors were obtained. Sperm and testis were prepared from Sprague Dawley rats (average age 10 weeks). Rat testis tissue pieces were embedded immediately after preparation in OCT Tissue-Tek and plunge-frozen in a mixture of isobutanol and dry ice followed by cryosectioning. For whole-mount immunofluorescence microscopy, sperm were prepared from testis and epididymal tissue, washed in PBS, mounted, processed and fixed on poly-l-lysine-coated slides as described previously [56] . Immunofluorescence microscopy Immunofluorescence microscopy was performed as described before [57] . Cryosections were thawed at room temperature and fixed with 2% paraformaldehyde for 5 min. After washing with PBS, the sections were incubated for 2 h with PBS containing 0.5% Triton X-100 and 10% goat serum (PBS/T/S) at room temperature. Incubation with the primary antibodies (diluted in PBS/T/S) was done overnight at 4 °C. The sections were then washed four times for 10 min with PBS before incubation with the secondary antibodies (diluted in PBS/S without Triton X-100) for 1 h at room temperature. The sections were incubated for 3 min with 1 μg ml −1 4',6-diamidino-2-phenylindole dihydrochloride, washed four times for 10 min with PBS and two times shortly with water before mounting with Mowiol containing 2 mg ml −1 p-phenylenediamine. For cytological overviews of haematoxylin-stained sections, a X20 0.8 numerical aperture PlanApochromat objective was used on a Zeiss Axioplan II microscope with the colour camera AxioCam HRC. For high-resolution immunofluorescence imaging, the X100 PlanApo 1.4 numerical aperture oil immersion objective was used on a Zeiss Imager Z1 microscope and Zeiss LSM700 laser scanning confocal microscope. Image capture for immunofluorescence microscopy was carried out with the AxioCam MRM b/w camera using the Axiovision or ZEN software. Image processing and annotation was done with Adobe Photoshop, Adobe Illustrator and ImageJ ( http://rsbweb.nih.gov/ij/ ). Electron microscopy Cells grown on Thermanox plastic coverslips (Nunc). Seventy-two hours after knockdown, cells were washed with PBS and fixed for 30 min at room temperature with 2.5% glutaraldehyde in cacodylate buffer (50 mM cacodylate pH 7,4 and 50 mM NaCl). Cells were washed and post-fixed for 1 h at room temperature with 0.5% OsO 4 in cacodylate buffer. After washing with water, cells were incubated for 30 min with 0.1% tannic acid in 250 mM Hepes pH 7.4 followed by 2% uranyl acetate, 90 min at room temperature. Cells were dehydrated in a graded series of ethanol and embedded in Spurr’s resin (Ted Pella) [58] . Ultrathin sections (70 nm) were prepared with an ultramicrotome (Reichert Ultracut E; Leica) and mounted on pioloform-coated electron microscopy copper grids (200 mesh). Sections were counterstained with uranyl acetate and lead citrate for 20 s. Image acquisition was performed on a Philips CM100 TEM. For pre-embedding labelling, samples were fixed in methanol at −20 °C, labelled with primary LGALS3BP or negative control antibody (non-specific rabbit IgG; Jackson Immunochemicals), washed, detected with secondary antibodies (anti-rabbit, conjugated to 10 nm gold; British BioCell), washed, post-fixed in glutaraldehyde and processed as described above. Immunogold labelling on pre-fixation-extracted U2OS cells was carried out as for immunofluoresence microscopy. Fixation and embedding was carried out as described above. Post-embedding labelling using London Resin (LR)-gold was carried out as described before [59] . Flow cytometry Fixation and propidium iodide staining of U2OS cells was performed according to the standard protocols (Current Protocols in Cell Biology, Cell Cycle Analysis 8.4.3). Cells were fixed in ice-cold 70% ethanol overnight and stained with propidium iodide staining solution (50 μg ml −1 pancreatic RNaseA (Sigma) and 50 μg ml −1 propidium iodide (Calbiochem) in PBS) for 1.5 h at 37 °C. The DNA content was quantified on a flow cytometer (BD FACSArray Bioanalyzer System; BD Biosciences) and analysed using FlowJo software (Tree Star). The cell populations were gated and quantified within the different cell-cycle phases. RT–PCR of tissue samples RNA was extracted from tissues after verification of tumour status using TRIZOL reagent (Invitrogen). RNA quantity was measured by NanoDrop (Peqlab), and RNA quality was assessed with the Experion system (Bio-Rad). Only samples with clear peaks for 18/28s rRNA were included in the analysis. A total of 10 μg RNA was reverse transcribed using the High Capacity cDNA Synthesis Kit (Applied Biosystems) and quantitative PCR was performed using the Power SYBR Green Mastermix (Applied Biosystems) in a 10 μl volume in 384 well plates. Liquid handling was done by a Hamilton Starlet Pipetting station, and PCR was performed on Applied Biosystems 9700 Gene Analyzers in triplicates. Primers for all genes are intron-spanning and were designed using open source PerlPrimer software (Marshall, 2004). Raw Ct values were exported, triplicates were collated as median, the relative expression was calculated for each sample using glyceraldehyde-3-phosphate dehydrogenase as a housekeeping gene and normalized to a tissue pool sample. Because of the small amount of glandular tissue in normal breast samples, fibroadenoma of the breast was used as control, and for similar reasons, cystadenome/borderline was used as control tissue in the ovary. A dditional information How to cite this article: Fogeron, M-L. et al . LGALS3BP regulates centriole biogenesis and centrosome hypertrophy in cancer cells. Nat. Commun. 4:1531 doi: 10.1038/ncomms2517 (2013).